Morphological and genetic evidence for early Holocene cattle management in northeastern China The domestication of cattle is generally accepted to have taken place in two independent centres: around 10,500 years ago in the Near East, giving rise to modern taurine cattle, and two millennia later in southern Asia, giving rise to zebu cattle. Here we provide firmly dated morphological and genetic evidence for early Holocene management of taurine cattle in northeastern China. We describe conjoining mandibles from this region that show evidence of oral stereotypy, dated to the early Holocene by two independent 14 C dates. Using Illumina high-throughput sequencing coupled with DNA hybridization capture, we characterize 15,406 bp of the mitogenome with on average 16.7-fold coverage. Phylogenetic analyses reveal a hitherto unknown mitochondrial haplogroup that falls outside the known taurine diversity. Our data suggest that the first attempts to manage cattle in northern China predate the introduction of domestic cattle that gave rise to the current stock by several thousand years. The domestication of animals represents one of the most important achievements in human history during the last 15,000 years [1] , [2] and, by supporting high local population densities, it is considered a key prerequisite for the development of human civilization. Among the four major Old World livestock species (cattle, goats, sheep and pigs), cattle are arguably the most important one: cattle provide meat, milk, hides for leather, and draught force for pulling carts, ploughing and other tasks [3] . On the basis of archaeological data and genetic analyses, the current consensus, albeit sometimes disputed, is that domestication of aurochs took place independently in two different geographical regions, the Near East and South Asia. Cattle domestication in the Near East is thought to have taken place around 10,500 years BP (before present), giving rise to taurine cattle ( Bos taurus [4] , mainly mitochondrial haplogroup T), whereas domestication in southern Asia has been dated later to about 8,500 years BP resulting in modern zebu (indicine) cattle ( B. indicus [5] , mitochondrial haplogroup I). Although the vast majority of modern cattle carry mitogenomes belonging to haplogroups T and I, several additional haplogroups (Q, P and R, all being phylogenetically closer to T than to I) have been identified. Haplogroup P was the most common haplogroup in European aurochs and has so far been identified in only two modern cattle [6] , [7] . Its occurrence in the modern cattle gene pool is generally explained by rare introgression events between female European aurochs and domesticated cattle introduced from the Near East [8] . Haplogroup Q is relatively close to haplogroup-T sequences and has been suggested to have entered the cattle mitochondrial DNA (mtDNA) gene pool during the initial domestication process in the Near East [9] . In contrast, haplogroup R is phylogenetically very distinct from P, Q and T and has so far only been found in modern Italian cattle [9] . As haplogroup P, it most probably represents a remnant of introgression from wild aurochs into the early domestic cattle gene pool. Finally, another haplogroup, E, was identified from several aurochs specimens from Europe [7] , [10] , but has to date not been detected in modern domesticated cattle. In summary, like other domesticated animal and plant species (reviewed in ref. 11 ), cattle domestication was a complex process and it is likely that additional details of this process remain to be revealed. Here we provide multidisciplinary evidence for management of cattle populations in northern China around 10,660 years ago, contemporary with the first domestication of cattle in the Near East. We describe a bovid mandible that was discovered in northeast China and dated to ~10,660 years BP. The specimen displays hyperattrition on the last premolar and first molar of both halves of the mandible, which is best explained by long-term human management. Ancient DNA analyses show that the individual did not belong to the same bovid mitochondrial lineages that have been domesticated in the Near East and South Asia. The combination of its age, attrition pattern and genetic signature suggests that this specimen represents the earliest evidence for cattle management in northeast China. Carbon dating of the specimen In 2005, a well-preserved complete bovid mandible was discovered from the Kongni ditch (45° 53" N, 125° 55" E), 48 km NWW of Harbin in northeastern China ( Fig. 1 ). From the discovery context, the age of the cattle specimen was estimated to be Late Pleistocene. Two subsamples of bone from the cattle mandible were sent to two different laboratories for radiocarbon dating: the Leibniz Laboratory for Radiometric Dating and Stable Isotope Research in Kiel (Germany) and the Joint Laboratory of accelerator mass spectrometry (AMS) Radiocarbon Dating, run by the School of Archaeology and Museology and the School of Physics, Peking University, China. Both laboratories carried out the entire dating process independently, including sample pretreatment, gelatine extraction, graphite preparation and AMS radiocarbon measurement. The C:N ratio of the extracted gelatine (2.878; Supplementary Table S1 ) falls into the range of 2.8–3.5, demonstrating the high quality of the extracted protein [13] . The δ 13 C values of gelatine and radiocarbon dates from the two laboratories match closely, further validating the reliability of the results. The AMS 14 C dates determined in the two laboratories are 10,756–10,565 and 10,758–10,565 calibrated years BP (95.4% probability; see also Supplementary Table S1 ), respectively, placing the specimen firmly at the beginning of the Holocene. 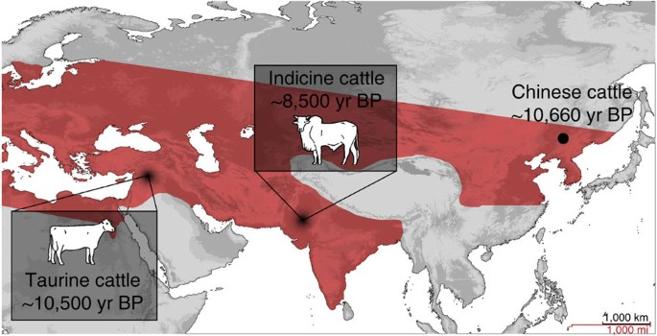Figure 1: Locations of cattle domestication centres compared with aurochs distribution. Map indicating the proposed centres and ages of taurine and indicine cattle domestication, relative to the Chinese specimen investigated in this study. The distribution of aurochs (Bos primigenius) is displayed in red (after ref.12), showing the presence of aurochs in the region where the proposed cattle management took place. Figure 1: Locations of cattle domestication centres compared with aurochs distribution. Map indicating the proposed centres and ages of taurine and indicine cattle domestication, relative to the Chinese specimen investigated in this study. The distribution of aurochs ( Bos primigenius ) is displayed in red (after ref. 12 ), showing the presence of aurochs in the region where the proposed cattle management took place. Full size image Morphological characteristics The specimen consists of conjoining left and right mandibles, with full tooth rows from the second premolar to the third molar (that is, P2–M3; Supplementary Fig. S1 ) on both mandibles. Both the specimen’s overall morphology and detailed morphology of the molar teeth allow confident attribution to Bos, rather than Bison or other large selenodont mammals. The specimen is from a mature individual with marked attrition on all molars and premolars. Dentine exposure extends across the full occlusal surface of M3, and exposure on the M3 hypoconulid is confluent with that on the more mesial parts of the tooth, a feature indicative of advanced attrition and thus a relatively advanced age [14] . The mandible exhibits exceptional attrition affecting the mesial half of M1 and the distal one-third of the adjacent P4. In this region, the mandibular occlusal plane (that is, the ‘chewing surface’ of the teeth) is sharply concave, deviating by 7–8 mm from the gentle curve of the occlusal plane ( Fig. 2 , Supplementary Fig. S1 ). This localized hyperattrition is bilateral, and developed to a closely similar extent on both mandibles. On the buccal aspect of the left mandible, there is an area of reactive periostitis that extends along the alveolar margin from the distal edge of P3 to the distal edge of M1, indicating long-term repetitive stress on this particular region of the mandible. Radiographs ( Fig. 2 , Supplementary Fig. S2 ) show root and alveolar bone development in the region of hyperattrition to be normal, ruling out any developmental causes for the observed hyperattrition. Therefore, we propose that these morphological features most probably indicate intensive oral stereotypy caused by human management of the individual in question (see Discussion for further details). 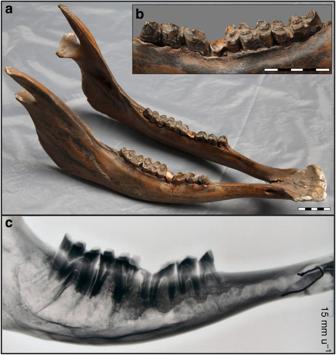Figure 2: Early-Holocene cattle mandible discovered in northeast China. Different views of the mandibles found at Kongni ditch, northeastern China, showing bilateral and symmetrical overattrition of M1 (a). An area of periostitic reaction can be seen adjacent to P4 and M1 on the buccal aspect of the left mandible (b). Radiographs of right mandible indicate normal root and alveolar bone development (c). Scales foraandbare given in centimetres. Figure 2: Early-Holocene cattle mandible discovered in northeast China. Different views of the mandibles found at Kongni ditch, northeastern China, showing bilateral and symmetrical overattrition of M1 ( a ). An area of periostitic reaction can be seen adjacent to P4 and M1 on the buccal aspect of the left mandible ( b ). Radiographs of right mandible indicate normal root and alveolar bone development ( c ). Scales for a and b are given in centimetres. Full size image Analysis of ancient mtDNA As modern cattle mtDNA diversity has been intensively studied, we analysed mtDNA sequences of the Chinese specimen to place it within the currently known genetic variability of modern and ancient bovids and to determine whether it belongs to any known domestic cattle haplogroup. We first amplified a 159-bp (including primers) fragment of the cattle mitochondrial D-loop region from both DNA extracts to verify the success of the extraction, as well as to obtain a preliminary indication of the phylogenetic position of the specimen ( Supplementary Methods , Supplementary Table S2 , Supplementary Fig. S3 ). The retrieved sequence has not been described before, and its phylogenetic position within the network suggested that it is phylogenetically distinct from all bovine haplogroups described to date. Because of the problems associated with the analysis of short mtDNA fragments only [15] , [16] , we then used DNA hybridization capture to target the full mitogenome of the specimen. We extracted DNA from two subsamples of the mandible (bone as well as tooth), using standard ancient DNA protocols [17] and precautions [18] . The extracts were built into Illumina sequencing libraries according to the protocol in ref. 19 . To enrich the libraries in endogenous DNA content, we used a modified hybridization capture protocol based on the protocols in refs 20 , 21 , 22 that uses biotinylated DNA baits to capture the desired sequences. We used European bison DNA for construction of the baits so that endogenous sequences and potential post-capture PCR artefacts (chimeras) would be distinguishable during the analysis stage ( Supplementary Methods , Supplementary Table S3 ). The enriched libraries were sequenced on a single Illumina HiSeq2000 lane, yielding a total of 88,061,646 reads, of which 3,801 unique sequence reads mapped to bovid mitogenomes (see Methods, Supplementary Methods , Supplementary Tables S3–S5 ). Mitochondrial reads exhibited DNA damage patterns typical of post-mortem depurination and cytosine deamination ( Supplementary Methods , Supplementary Fig. S4 ), suggesting that the sequence data originated from ancient DNA templates. In addition, we screened mitochondrial sequence reads at sites specific for bison and the different mitochondrial taurine haplogroups to estimate maximum contamination levels. We note that at such sites, post-mortem DNA damage resulting in nucleotide misincorporation as well as sequencing errors could transform genuine endogenous alleles into contamination-like alleles. Therefore, our approach is conservative and provides maximal contamination estimates. We found potential contaminant alleles 15 times at such sites, suggesting an upper bound to contamination levels of around 5% ( Supplementary Methods , Supplementary Tables S6 and S7 ). Using a strict majority rule and a minimal depth-of-coverage of 2, we constructed a mitochondrial consensus sequence with 16.7-fold coverage, consisting of 94.3% (15,406 bp) of the mitogenome ( Supplementary Methods ). The consensus sequence of the Chinese specimen was aligned with 26 publicly available mitogenomes, including 14 taurine cattle ( B. taurus ) that cover all known haplogroups, except E, for which no complete mitogenome is available, 3 zebu ( B. indicus ), 3 yak ( B. grunniens ), 3 American bison ( Bison bison ) and 3 European bison ( B. bonasus ; Supplementary Table S8 ). Phylogenetic analyses place the Chinese cattle sequence together with taurine cattle sequences with 100% bootstrap support and a Bayesian posterior probability of 1. Within taurine cattle, it is supported as a sister group to the currently known variation of the taurine mtDNA sequences with lower (75%) bootstrap support in maximum likelihood analyses ( Fig. 3 ), but forms an unresolved trichotomy with the superhaplogroup R and the rest of taurine cattle in both unpartitioned and partitioned Bayesian analyses ( Supplementary Fig. S5 ). A basal position is also the most highly supported by topology tests, but neither a sister group relationship between the Chinese cattle and the superhaplogroup R nor the trichotomy recovered in the Bayesian analysis can be rejected with statistical significance ( Supplementary Table S9 , Supplementary Fig. S6 ). The phylogenetic results show that the Chinese cattle specimen unambiguously belongs to the taurine cattle group but represents a hitherto unknown divergent mitochondrial haplogroup, in line with its geographically distinct origin. This interpretation is also supported by a phylogenetic network based on the ~60% (519 bp) of the mtDNA control region retrieved with the hybridization capture approach ( Supplementary Methods , Supplementary Fig. S7A ). An additional network spanning a total of 412 bp of cytochrome B and control region indicates that the Chinese cattle is also genetically distinct from the enigmatic haplogroup E ( Supplementary Methods , Supplementary Fig. S7B ) [7] , [10] . Although it is currently only represented by a single sequence, because of its phylogenetic distinctness, we have decided to assign it to a new haplogroup, termed haplogroup C, acknowledging its geographical origin ( Supplementary Table S5 ). 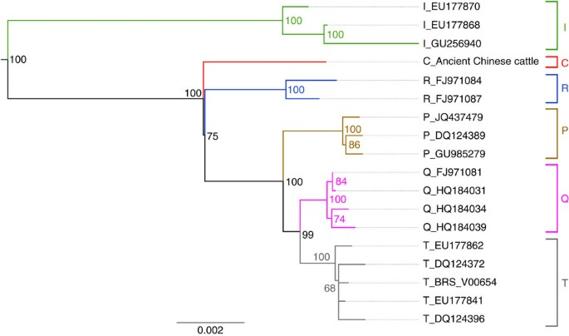Figure 3: Phylogeny of ancient and modern cattle mitogenomes. Phylogenetic tree of the investigated taurine and zebu cattle mitogenome sequences together with the sequence obtained from the Chinese specimen. The tree was rooted with 6 Yak (Bos grunniens) sequences. Letters to the right indicate the commonly accepted taurine cattle haplogroups, that is, the vastly predominant T and Q plus the very rare, more divergent P and R clades. Numbers indicate maximum likelihood node support after 100 bootstrap replicates. Figure 3: Phylogeny of ancient and modern cattle mitogenomes. Phylogenetic tree of the investigated taurine and zebu cattle mitogenome sequences together with the sequence obtained from the Chinese specimen. The tree was rooted with 6 Yak ( Bos grunniens ) sequences. Letters to the right indicate the commonly accepted taurine cattle haplogroups, that is, the vastly predominant T and Q plus the very rare, more divergent P and R clades. Numbers indicate maximum likelihood node support after 100 bootstrap replicates. Full size image Although northern China has been discussed as a centre of domestication for millet [23] , [24] and pigs [25] , [26] , there has so far been no evidence of autochthonous cattle domestication in this region. The specimen investigated in this study clearly derives from an animal belonging to the Bos taurus/indicus group and shows exceptional attrition affecting the mesial half of M1 and the distal one-third of the adjacent P4. Two possibilities should be considered as potential causes of this feature. First, overeruption of the maxillary M1 could produce the observed localized attrition, by bearing heavily on the corresponding mandibular M1. However, this is highly unlikely to have occurred both bilaterally and symmetrically. Second, the observed attrition could have been caused by habitual chewing of some hard object that extended across the width of the mouth, limited to the mesial part of M1 by the cheeks. For example, an elongated object held against the ‘corners’ of the mouth would tend to be located at the point of the observed heavy attrition. The repeated chewing of hard objects, known as bar-biting or crib-biting, is most commonly seen in horses [27] . Bar-biting and other abnormal oral behaviours (or normal behaviours at abnormal frequencies) are also seen in cattle when the ‘wild’ pattern of ad lib grazing in a social group is disrupted [28] , [29] , [30] , and particularly when animals are tethered or penned [31] . Therefore, we suggest that the attrition seen on this specimen indicates repeated and intensive stereotypy, consistent with a long-term disruption to the animal’s dietary and social welfare, most probably caused by some degree of human management of the cattle population of which this individual was a part. We do not suggest that the hyperattrition was caused by a form of harness or restraint, but by habitual chewing of elongated objects, such as pieces of wood, by this animal over a considerable period of time. These behavioural traits are seen in modern domestic cattle, many generations removed from the ‘wild’, and so seem likely to have been at least as frequent in the first cattle herds that were isolated and managed by people. The apparent absence of other published archaeological records for bar-biting in cattle may reflect a lack of recognition of the condition, not least because cattle mandibles are rarely encountered as conjoined pairs. It may also reflect a higher probability of mismanagement of animals during the early stages of domestication because of unfamiliarity with the species’ behaviour leading to significant trauma and behavioural anomalies. However, although evidence for bar-biting has so far not been reported for cattle in archaeological records, overattrition of M1 and the adjacent P4 is seen in domestic pigs, including archaeological specimens ( Supplementary Fig. S8 ). In this case, the cause is also assigned to stereotypic behaviour by a stressed or bored animal [32] . The Chinese specimen therefore suggests human management of cattle in northeastern China, predating the currently accepted evidence of domestic cattle in this region (4,000–5,000 BP [33] ) by several thousand years and being as early as the initial domestication of taurine cattle in the Near East between ca. 11,000 and 10,000 BP (ref. 4 ). The degree of hyperattrition of the M1 observed for the investigated specimen together with the evidence for advanced age at the time of death of the animal (~7–9 years) suggest that the animal from which the mandible originates was under human management for an extended time period, potentially from birth or through taming when young. Whether management that results in changes to feeding and behavioural stereotypy represents domestication is a matter of semantics beyond the remit of this paper. However, it should be noted that scientific discoveries during the last decade have shown that animal as well as plant domestications represent extended processes rather than sudden events [11] , [34] , [35] , [36] , [37] . For example, it has been argued that canid remains being as old as ~30,000 BP may represent the remains of early dog domestication attempts (refs 38 , 39 , 40 , 41 but see refs 42 , 43 ). Moreover, it has been suggested that at least some domesticated species (for example, dogs, cats and pigs) underwent an extended phase of commensalism with humans before domestication [35] , [37] . Finally, humans likely managed at least some animal populations before they eventually domesticated them [44] . Altogether, there is an emerging consensus that the domestications of both animals and plants represent complex processes, including pre-domestication management of (semi-) wild populations, commensalism and multiple, sometimes failed domestication attempts, including on species that were later and/or somewhere else successfully domesticated [11] , [34] . The distinct phylogenetic signal of the Chinese cattle specimen suggests that it belonged to a distinct mitochondrial population rather than to the populations that were domesticated in the Near East (haplogroup T) or in the Ganges Valley (haplogroup I). Theoretically, this result could be explained by introgression of mtDNA from a local wild population into T-haplogroup cattle imported from the Near East. However, given that the investigated specimen dates to the same time when cattle domestication started in the Near East, this explanation seems rather unlikely. Therefore, the morphological and genetic data together with precise dating of the specimen provide substantial evidence that people were managing genetically distinct, and therefore probably locally originating, taurine cattle in northeastern China at least 10,660 year ago, causing sufficient impact on their social behaviour to lead to oral stereotypies with some animals. This is an unexpected result, given the current focus on early domestication of taurine cattle in the Near East and Zebu cattle in southern Asia. Intriguingly, recent studies have found evidence for millet domestication from the same area dating back to 11,000 years BP [23] , [24] . Moreover, it has been argued that the same region represents one of several areas of early pig domestication, dating to at least 8,500 years BP but probably earlier [25] , [26] . Although this is currently largely speculative, the coincidence in time and place of millet-based agriculture, management of cattle and possibly pig domestication, together with the putative origin of modern domestic dogs [43] , [45] not far south, raises the possibility that we are seeing evidence of what might have been one of the earliest mixed agricultural complexes in the world. The haplogroup retrieved has so far not been found in modern cattle. However, as mtDNA represents a single genetic locus, it is prone to genetic drift and could easily have been lost by drift even if hybridization between the population to which the Chinese specimen belonged and other domesticated cattle populations has occurred. Further analyses on nuclear DNA will be necessary to show whether this early Chinese cattle management was a short-lived episode or whether it has contributed to the nuclear gene pool of modern cattle. DNA extraction We extracted DNA from one tooth and one bone sample, both obtained from drilling into the original specimen (York laboratory numbers 2458 and 2459, respectively), using a silica-based extraction protocol following ref. 17 . All procedures were performed in a dedicated ancient DNA laboratory at the University of York, with appropriate contamination precautions in place [18] . One extraction blank (mock extraction) was included and treated exactly as the extracts throughout the whole process. From the bone sample (2,458), 135 mg were used and from the tooth sample (2,459), 97 mg were used for extraction. Library preparation Next-generation sequencing libraries for the Illumina platform were prepared from both extracts (bone and tooth), as well as from the mock extract and a water control, following ref. 19 , with some minor modifications as described below. The blunt-end repair reaction was performed in 35 μl reaction volume instead of 70 μl because of the limited volume of extract available (25 μl of ancient DNA (aDNA) extract were used as template). Between the different steps in library preparation, the samples were purified using Qiagen MinElute PCR purification columns according to the manufacturer’s instructions, with two elution steps each using 10 μl Qiagen EB buffer in each. Bait preparation and library enrichment We created biotinylated baits from modern mtDNA, according to a protocol adapted from refs 20 , 21 , 22 . To prevent any carry-over baits from interfering in downstream steps (by creating chimeras), baits were prepared to contain uracil and/or biotinylated uracil so that the baits can be digested after hybridization capture (see Supplementary Methods for more details on capture protocols). Indexing PCRs to create molecular barcoded libraries for the individual samples were performed in 50 μl reactions using the same master mix as described above and 10 amplification cycles (see Supplementary Methods for more details). Indexed libraries were pooled in equimolar amounts and sequenced on a single lane of an Illumina HiSeq2000 by Genterprise (Mainz, Germany). Sequence analysis and assembly A total of 88,061,646 single-end Illumina reads were trimmed for adapter sequences at their 3′-end following a pairwise alignment procedure and using the software AdapterRemoval available for download at http://www.code.google.com/p/adapterremoval/ (ref. 46 ). A minimal sequence identity of 90% over 5–10 nucleotides was required for adapter alignment (this threshold was lowered to 67% for alignments extending over 11 nucleotides). In addition, reads showing stretches of bases with low-quality scores and/or Ns at sequence ends were trimmed from the first nucleotide position showing the low-quality score. Reads starting with stretches of at least one undetermined base were trimmed, resulting in a final sequence starting at the first position showing a determined base. We next focused on reads showing a sequence length longer than 25 nucleotides after trimming to provide enough information for unambiguous mapping against reference mitogenomes (Accession numbers: JQ437479, Bos primigenius ; AF492350, B. indicus ; NC_014044, Bison bonasus ). As the mitogenome is circular, the first 30 nucleotides were manually duplicated at the end of the reference sequences to identify reads that would partially overlap the ends of the mitogenome sequence until a final consensus sequence was called. Filtered and trimmed reads originating from different DNA libraries were processed separately until the final mitochondrial consensus sequence was generated. Burrows–Wheeler Aligner [47] was used for mapping using default parameters, except that the seed was disabled following the recommendations from ref. 48 . Reads were filtered for mapping quality scores higher than 30 and for mapping unique positions. The 5′-coordinates of read alignments on the mitogenome were used to remove PCR duplicates as implemented in MarkDuplicates from Picard tools ( http://www.picard.sourceforge.net ). We found that a larger number of sequence reads could be aligned to the B. primigenius mitochondrial reference genome. Therefore, sequence reads from final BAM files resulting from mapping against the B. primigenius mitochondrial reference genome were recovered and converted to fasta format before pairwise realignment was performed using Muscle [49] . A subset of reads was identified only when the mitogenomes of B. indicus and/or B. bonasus were used as reference. Those reads probably originated from mitochondrial regions where the sample was more distant to the B. primigenius reference and were added to the multifasta alignment. A final alignment was generated using read alignments from each DNA library (for a total of 3,801 sequence reads) and a final consensus was called using a strict majority rule and requiring a minimum base coverage of 2. The polymorphic positions compared with the Bovine Reference Sequence (Genbank Accession number V00654) are listed in Supplementary Table S5 . DNA fragmentation and nucleotide damage patterns were analysed using the mapDamage [50] package and BAM files generated following mapping against the B. primigenius mitochondrial reference genome ( Supplementary Fig. S5 ). Finally, we verified that our final consensus sequence did not consist of numts by translating the 13 protein-coding genes into protein sequences using the vertebrate mitochondrial code. No premature stop codon was observed, suggesting that the final consensus sequence consists of functional gene elements and not pseudogenes. Annotation of the mitogenome was performed using MITOS [51] . Phylogenetic analyses of mitogenomes We downloaded 26 complete mitogenome sequences from Genbank, which were selected for encompassing the whole spectrum of the known mitochondrial diversity so far reported within Bos taurus, Bos indicus and Bos gruniens , as well as within Bison bison and Bison bonasus ( Supplementary Table S8 ). Whole mitogenomes were aligned manually using Seaview v4 (ref. 52 ), and sequences coding for the 13 proteins and 2 ribosomal RNAs were extracted and merged within a single alignment that we used for phylogenetic analyses. The final alignment represents 13,945 nucleotides of the Bovine Reference Sequence (Accession number V00654). We performed two types of analyses: unpartitioned and partitioned according to first, second and third codon positions of the protein codon regions, 12S rRNA and 16S rRNA. The best substitution models were selected in jModeltest v0.1.1 (ref. 53 ) for each of the analyses. For the unpartitioned analysis, we selected GTR+G+I as the best substitution model running jModeltest v0.1.1 (ref. 53 ) on the BioNJ topology and using the corrected Akaike Information Criterion. Likelihood phylogenies were constructed using PhyML v3.1 (ref. 54 ) and node support was evaluated through the approximate likelihood ratio test (SH-like) and 100 bootstrap pseudoreplicates. Bayesian phylogenies were reconstructed using MrBayes [55] , [56] on the one hand (20 million generations, two runs of four chains each, sampling every 1,000 generation and discarding the first 25% generations as burnin) and BEAST [57] on the other hand. For BEAST, we constrained the main clades consistently identified with PhyML and MrBayes as monophyletic. The time to the most recent common ancestor of those clades was estimated assuming a strict clock and using the Yule speciation model, as our alignment consisted of individuals from different species. BEAST was run for 50 million generations sampled every 1,000 generations. Convergence was checked using Tracer v1.5 (available from http://www.beast.bio.ed.ac.uk/Tracer ) and the time to the most recent common ancestor posterior distributions were calculated after discarding the first 25% generations sampled as burnin. We considered as possible calibration points the three dates reported in ref. 15 for the divergence between Bos taurus and Bison bison ( Supplementary Table S10 ). In the partitioned analyses, the best substitution models were selected in jModeltest v0.1.1 (ref. 53 ) using the Bayesian information criterion and implemented in the Bayesian phylogenetic analyses as described above. The resulting phylogenetic tree is displayed in Supplementary Fig. S6 (see Supplemetary Methods for more details). Accession codes : The taurine mitochondrial DNA genome sequence generated from the fossil mandibles described in this study is deposited in GenBank nucleotide database under accession number KF525852 . How to cite this article: Zhang, H. et al. Morphological and genetic evidence for early-Holocene cattle management in northeastern China. Nat. Commun. 4:2755 doi: 10.1038/ncomms3755 (2013).